Unreachable glass transition in dilute dipolar magnet In magnetic systems the combined effects of disorder and frustration may cause the moments to freeze into a disordered state at a spin-glass transition. Recent experiments have shown that the rare earth compound LiHo 0.045 Y 0.955 F 4 freezes, but that the transition is unreachable because of dynamics that are 10 7 times slower than in ordinary spin-glass materials. This conclusion refutes earlier investigations reporting a speed-up of the dynamics into an exotic anti-glass phase caused by entanglement of quantum dipoles. Here we present a theory, backed by numerical simulations, which describes the material in terms of classical dipoles governed by Glauber dynamics. The dipoles freeze and we find that the ultra-slow dynamics are caused by rare, strongly ordered clusters, which give rise to a previously predicted, but hitherto unobserved, Griffths phase between the paramagnetic and spin-glass phases. In addition, the hyperfine interaction creates a high energy barrier to flipping the electronic spin, resulting in a clear signature in the dynamic correlation function. The rare-earth compound LiHo 0.045 Y 0.955 F 4 has been used in studies of such varied phenomena as quantum phase transitions [1] , random field physics [2] , persistent coherent oscillations [3] , quantum annealing [4] , quantum tunnelling [5] and entanglement [6] (for a review of LiHo x Y 1− x F 4 , see ref. 7 ). This, despite the fact that the parent compound, LiHoF 4 , is one of the best realisations of the (dipolar) Ising model [8] , [9] , [10] , one of the most fundamental models in condensed matter physics. The magnetic properties arise from the Ho 3 + ions decorating a tetragonal lattice. Hund's rules dictate a 17-fold degenerate 5 I 8 ground state, but the crystal field lifts the degeneracy and forces the angular momentum to point along the c axis (with a moment of 6.9 μ B ), resulting in a two-state Ising model, where the dipolar coupling constant J d =0.214 K. LiHoF 4 is a dipolar ferromagnet with a transition at T c =1.5 K. Random disorder can be induced in this inherently frustrated dipolar model by substituting non-magnetic yttrium for magnetic holmium, yielding LiHo x Y 1− x F 4 . This suppresses the ferromagnetic transition, which finally vanishes around x =0.25. Early studies indicated that at intermediate dilution ( x =0.167) χ ″( ω ) broadened in a traditional spin-glass fashion, whereas in the limit of extreme dilution ( x =0.045) χ ″( ω ) became narrower as the temperature was lowered. This led to the conclusion that the material behaves as an exotic spin-liquid (anti-glass), supporting coherent oscillations at extreme dilution, whereas it is a traditional spin glass at intermediate dilution [11] , [3] , [6] . Measurements by a different group led to the conclusion that there is no spin-glass freezing at any temperature [12] . More recently, a careful re-investigation of the dynamic susceptibility covering more than six decades in frequency at x =0.045 did not reveal the previously observed narrowing of the spectral density [13] Instead, χ ″( ω ) appeared to broaden in a normal spin-glass fashion also in the limit of extreme dilution. Furthermore, the characteristic relaxation time was found to follow a conventional power-law scaling, τ ~ τ 0 |( T − T c )/ T c | − vz . This led to the conclusion that the finite-temperature glass phase extends all the way to x =0. However, the dynamics was found to be surprisingly slow, with an intrinsic time scale of τ 0 =16 s (commonly τ 0 ~10 −6 to 10 −7 s), limiting the measurements to T >1.8 T c . From a theoretical point of view, the model in equation (1) is expected to support a finite-temperature spin-glass phase extending to x =0 [14] , and recent Monte Carlo simulations, where the dynamics was sped up using a parallel tempering method, support this scenario [15] . To shed more light on this controversial low-temperature state, we scrutinise the dynamics of LiHo 0.045 Y 0.955 F 4 . In particular, we calculate the dynamic spin-correlation function C ( t )= M (0) M ( t ) , where M ( t ) is the time-dependent magnetisation of the system. Although this quantity is of central importance in many theoretical descriptions and simulations of spin glasses [16] , [17] , [18] , [19] , we are only aware of one experimental determination of C ( t ) in the critical spin-glass regime [20] . The difficulty is that low-noise experimental data covering many orders of magnitude in frequency is necessary for a reliable calculation. Fortunately, data of this kind is now available for LiHo 0.045 Y 0.955 F 4 (ref. 13 ). Dynamic correlation function We calculate C ( t ) using the fluctuation-dissipation theorem, The transformation is much facilitated by an analytic expression for the susceptibility. However, the most widely used Cole–Cole, Davidson–Cole and Havriliak–Negami functions [21] fail to capture the tails of the data at low temperatures [13] . Therefore, we propose the following functional form for the AC susceptibility: where the position and sharpness of the maximum are given by τ and n , whereas χ ″ vanishes with exponents α 1 , and α 2 . As Fig. 1 shows this form matches the data well, except for in the high-temperature, high-frequency tail, where the difference is most likely caused by a minor high-frequency phase shift in the susceptometer (J. A. Quilliam and J. B. Kycia, private communication). 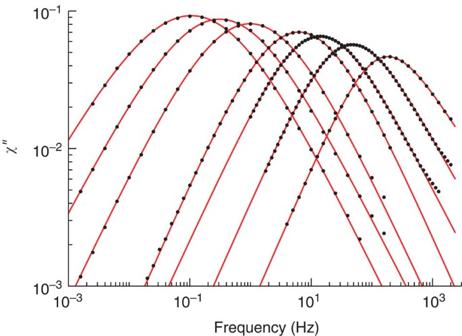Figure 1: Experimental out-of-phase susceptibility in LiHo0.045Y0.955F4. The experimental data (black dots) are from Quilliamet al.13, whereas red lines are best fits to equation (3) at temperatures 0.10, 0.11, 0.12, 0.14, 0.15, 0.17 and 0.20 K from left to right. Figure 1: Experimental out-of-phase susceptibility in LiHo 0.045 Y 0.955 F 4 . The experimental data (black dots) are from Quilliam et al . [13] , whereas red lines are best fits to equation (3) at temperatures 0.10, 0.11, 0.12, 0.14, 0.15, 0.17 and 0.20 K from left to right. Full size image Next, we calculate the dynamic magnetisation correlation function C ( t ) using equation (2). If LiHo 0.045 Y 0.955 F 4 were to undergo a traditional finite temperature spin-glass transition, we could expect a short-time algebraic decay, followed by a long-time stretched-exponential decay, C og ( t )=exp(− t / τ ) β / t α . This Ogielski form has been observed in Monte Carlo simulations of non-dilute Ising spin glasses, both in the nearest neighbour [18] and Sherrington–Kirkpatrick Ising models [19] . Furthermore, the only experimental determination of C ( t ) we are aware of also recovered C og ( t ) for the three-dimensional (3D) short-range spin-glass Fe 0.5 Mn 0.5 TiO 3 , using an approximate phenomenological relation C app ( t )=1− χ ′( t =1/ ω )/ χ ′( ω =0) (ref. 20 ). In Fig. 2 , we display the transformation of the experimental data using equation (2). Interestingly, we find that the Ogielski functional forms appear in reverse order compared with traditional finite temperature spin glasses. The short-time correlations are well described by a stretched exponential form ( C og ( t ) with α =0, red lines), whereas the long-time low-temperature decay is very close to algebraic, as indicated by the almost straight lines in the log–log plot. We have also applied the approximate method [20] ( C app ( t ), dotted blue line) and note that it agrees well qualitatively with the exact transformation as the temperature is lowered. 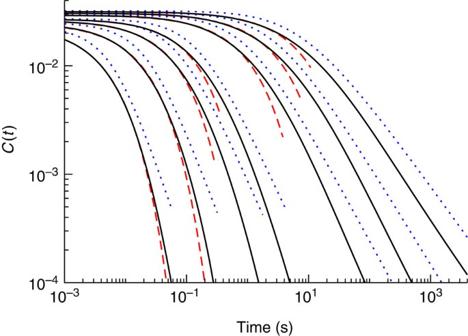Figure 2: Decay of correlations from experiments. C(t)determined from equation (2) (solid black lines) along with a fit to a stretched exponential form (Cog(t) witha=0, dashed red curves) and approximate calculation (Capp(t), doted blue lines). Temperatures are 0.20, 0.17, 0.15, 0.14, 0.12, 0.11 and 0.10 K from left to right. Figure 2: Decay of correlations from experiments. C(t) determined from equation (2) (solid black lines) along with a fit to a stretched exponential form ( C og ( t ) with a =0, dashed red curves) and approximate calculation ( C app ( t ), doted blue lines). Temperatures are 0.20, 0.17, 0.15, 0.14, 0.12, 0.11 and 0.10 K from left to right. Full size image Griffiths phase Having established the functional form of C ( t ) from recent experiments, we now use a Monte Carlo method based on Glauber dynamics to calculate C ( t ) from equation (1). First, we demonstrate that the slow long-time, low-temperature decay we have found in the experimental data stems from rare-ordered clusters with very slow dynamics. Rare-ordered regions have been predicted to give rise to a sub-exponential decay bounded below by C ( t )=exp(− c ln t ) d /( d −1) for a d -dimensional short-range spin glass [16] . This prediction for an intermediate Griffiths phase between the paramagnetic and the spin-glass phases has not been observed previously in the 3D spin glasses. In Fig. 3 , we show the Monte Carlo results for C ( t ) for 92 ( L =8) and 180 ( L =10) spins at 4.5% dilution. Just as in the experimental result in Fig. 2 , we find a very slow, almost algebraic low-temperature long-time decay. To investigate the origin of the slow decay, we show C ( t ) for 96 separate realisations in Fig. 4a . We note a very broad distribution of correlation times and the typical decay (average of the logarithm of C ( t ), lower yellow line) is a stretched exponential at long times, whereas the average decay (upper yellow line) is dominated by very few configurations at long times and decays algebraically. In Fig. 4b , we analyse the disorder realisation that gives the dominating contribution (marked by a red line in Fig. 4a ) by plotting C ( t ) for each of the 92 spins. We find that six spins (red) dominate the long-time decay, and a number of additional blue, green and violet spins also display strong correlations. 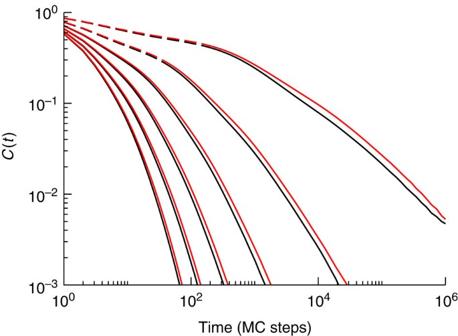Figure 3: Decay of correlations from simulations. Dynamic correlation function from Monte Carlo calculations forL=8 (black line) andL=10 (red line) at temperatures 0.35, 0.30, 0.25, 0.20, 0.15 and 0.10 K from left to right. The low-temperature initial algebraic decay is indicated by dashed lines. Figure 3: Decay of correlations from simulations. Dynamic correlation function from Monte Carlo calculations for L =8 (black line) and L =10 (red line) at temperatures 0.35, 0.30, 0.25, 0.20, 0.15 and 0.10 K from left to right. The low-temperature initial algebraic decay is indicated by dashed lines. 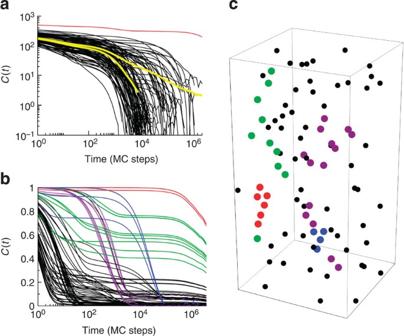Figure 4: Effects of strongly coupled clusters. (a) Dynamic correlation function for 96 separate disorder realisations. Thick yellow solid lines indicate typical decay (lower curve) and average decay (upper curve). For the topmost configuration (red line), the auto-correlation function for each individual spin is shown in (b). The colours of the auto-correlation functions mark clusters of spins, whose spatial positions are shown in (c). Full size image Figure 4: Effects of strongly coupled clusters. ( a ) Dynamic correlation function for 96 separate disorder realisations. Thick yellow solid lines indicate typical decay (lower curve) and average decay (upper curve). For the topmost configuration (red line), the auto-correlation function for each individual spin is shown in ( b ). The colours of the auto-correlation functions mark clusters of spins, whose spatial positions are shown in ( c ). Full size image To visualise these spins, we plot the spin configuration in Fig. 4c . We find that the red spins form a small ferromagnetic cluster elongated along the Ising direction. This constitutes a minimum energy configuration without frustration, as the dipolar interaction is ferromagnetic along the Ising direction. The red cluster is surrounded by a more diffuse green cluster, which also is elongated along the Ising direction. The blue spins form a small compact cluster, whereas the violet spins are near-neighbour pairs. Hence, the dynamic behaviour is dominated by rare strongly coupled clusters with long autocorrelation times. This is the signature of a Griffiths phase [22] . Because of the dilution and long-range interactions, the effect of these rare regions is much stronger in dilute dipolar models than in the short-range spin glasses. Hyperfine interaction Next, we focus on the short-time decay of C ( t ) in Fig. 3 . As in the previous spin-glass studies [18] , [20] , we find an algebraic decay at low temperatures (indicated by a dashed line). This differs from the experiments in Fig. 2 , where the decay is exponential at short times, indicating that the spins in the material are subject to an energy barrier not present in the simulation. A likely candidate is the relatively strong hyperfine interaction [23] , , where A =0.21 K and I z takes half-integer values between -7/2 and 7/2. We therefore include the hyperfine interaction and the relatively weak exchange interaction ( , with J e =0.12 K) in our simulation and show the results in Fig. 5 . The Monte Carlo results now agree well with the experiment, and both sets of curves exhibit exponential decay at short times and much slower decay, which approaches algebraic in the low-temperature, long-time limit. The inset displays the correlation time τ defined by C ( τ )=0.1 C (0), and this shows that the experimental relaxation time diverges slightly faster than the relaxation obtained from simulations. For the four lowest temperature, we also fit the experimentally determined relaxation to the form C ( t )= A exp(− c (ln ( t/t 0 )) 3/2 ) predicted for a 3D short-range spin glass [16] . We have not modified this expression to take the dipolar interaction into account, and we do not expect this functional form to accurately describe the initial decay. However, as is evident from Fig. 5 , it captures the slow-decaying tail rather well, giving further evidence to the existence of a Griffiths phase in LiHo 0.045 Y 0.955 F 4 . 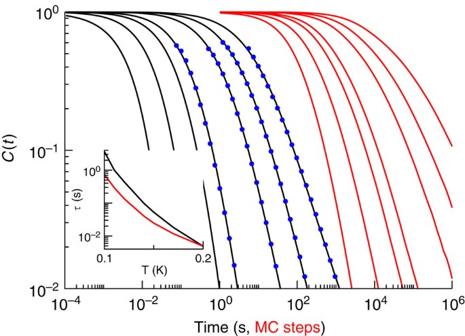Figure 5: Relaxation in LiHo0.045Y0.955F4. Dynamic correlation function for the experiments (black curves) compared with results of a Monte Carlo simulation (red curves), including dipolar, hyperfine and exchange interactions. The temperatures are 0.10, 0.11, 0.12, 0.14, 0.15, 0.17 and 0.20 K from right to left. Blue filled circles indicate a fit to the predicted formC(t)=Aexp(−c(ln (t/t0))3/2) (ref.16). The inset shows the corresponding correlation time as a function of temperature. The Monte Carlo correlation time has been rescaled to match experiments atT=0.2 K. Figure 5: Relaxation in LiHo 0.045 Y 0.955 F 4 . Dynamic correlation function for the experiments (black curves) compared with results of a Monte Carlo simulation (red curves), including dipolar, hyperfine and exchange interactions. The temperatures are 0.10, 0.11, 0.12, 0.14, 0.15, 0.17 and 0.20 K from right to left. Blue filled circles indicate a fit to the predicted form C ( t )= A exp(− c (ln ( t/t 0 )) 3/2 ) (ref. 16 ). The inset shows the corresponding correlation time as a function of temperature. The Monte Carlo correlation time has been rescaled to match experiments at T =0.2 K. Full size image Ultra-slow dynamics Finally, we show how the extremely slow relaxation time τ 0 =7.5×10 7 τ 1 =16 s found in Quilliam et al . [13] arises directly from the effects of the hyperfine interaction and strongly coupled clusters. Above the critical region, correlations decay exponentially, and we expect the Arrhenius scaling τ ( T )= τ 1 e Δ E / T to hold until collective effects change the scaling to τ ( T )= τ 0 |( T−T c )/ T c |− vz , which defines τ 0 = τ (2 T c ). Considering 2 T c at the edge of the critical region, we can estimate τ 0 as τ 0 = τ 1 e Δ E /2 Tc . In more ordinary spin-glass materials, Δ E and T c are both set by the same energy scale, namely the coupling constant J . Therefore, τ 0 and τ 1 are very close, s. In LiHo 0.045 Y 0.955 F 4 , on the other hand, T c is close to the mean-field value, K =0.0675 K, whereas Δ E is much larger because of the hyperfine interaction and strongly coupled clusters. From a best fit of to the Monte Carlo data in the inset of Fig. 5 , we obtain Δ E =1.56 K, which agrees remarkably well with the experimental result Δ E =1.57 K [13] . Using the experimental value [13] Tc =0.043 K, we obtain , which explains why τ 0 exceeds τ 1 so dramatically. In conclusion, we find that LiHo 0.045 Y 0.955 F 4 is well described by classical dipoles that freeze. The combined effects of the hyperfine interaction and strongly coupled clusters reverse the long- and short-time decay of C ( t ) compared with ordinary spin-glass transitions [18] , [20] . Furthermore, these effects cause τ 0 to exceed τ 1 by seven orders of magnitude. Remarkably, the glass transition is unaffected. The classical hyperfine interaction does not alter the transition, as the partition function factorises into an electronic and a nuclear part. The clusters, on the other hand, cannot destroy the phase transition, as the dimensionality of the cluster ( d =0) is less than the critical dimension [22] . Our results demonstrate the pervasiveness of the fluctuation-dissipation theorem and relaxational dynamics. The experimental measurements are very challenging because of the low temperatures and slow dynamics in the material, and we can only speculate that the previous observation of a spin-liquid phase (anti glass) may be because of difficulties with reaching equilibrium and cooling the sample. The present results may well pertain to other disordered dipolar-coupled materials, such as the rare-earth spin-ice materials, which support magnetic monopole excitations in their clean form. Numercial methods In the Monte Carlo simulation, we use periodic boundary conditions and the Ewald summation technique without a demagnetisation term to handle the long range of the dipolar interaction. The Monte Carlo cell is cubic with a linear size of L unit cells, containing 4× L 3 sites, of which a given percentage ( x ) are occupied by Ising spins. On average, one attempt to flip each spin is made during each Monte Carlo step. The update probability for each spin is given by the Glauber (heat-bath) algorithm P =(1+ e ΔE/T ) −1 , where Δ E is the energy change resulting from the attempted spin flip. Each disorder realisation is first equilibrated during 10 7 Monte Carlo steps using parallel tempering, followed by 10 8 Monte Carlo steps at fixed temperature during which the measurements are taken. The data shown in Figs 3 and 5 represents an average over 2,000 and 600 disorder configurations, respectively. How to cite this article: Biltmo, A. & Henelius, P. Unreachable glass transition in dilute dipolar magnet. Nat. Commun. 3:857 doi: 10.1038/ncomms1857 (2012).